Cyclin F suppresses B-Myb activity to promote cell cycle checkpoint control Cells respond to DNA damage by activating cell cycle checkpoints to delay proliferation and facilitate DNA repair. Here, to uncover new checkpoint regulators, we perform RNA interference screening targeting genes involved in ubiquitylation processes. We show that the F-box protein cyclin F plays an important role in checkpoint control following ionizing radiation. Cyclin F-depleted cells initiate checkpoint signalling after ionizing radiation, but fail to maintain G2 phase arrest and progress into mitosis prematurely. Importantly, cyclin F suppresses the B-Myb-driven transcriptional programme that promotes accumulation of crucial mitosis-promoting proteins. Cyclin F interacts with B-Myb via the cyclin box domain. This interaction is important to suppress cyclin A-mediated phosphorylation of B-Myb, a key step in B-Myb activation. In summary, we uncover a regulatory mechanism linking the F-box protein cyclin F with suppression of the B-Myb/cyclin A pathway to ensure a DNA damage-induced checkpoint response in G2. The DNA damage response serves to protect cells against DNA lesions from exogenous and endogenous sources. Following the detection of such lesions, cellular signalling stimulates DNA repair, cell cycle arrest and eventually senescence or apoptosis results if the DNA damage burden is massive. The cell cycle checkpoint in the G2 phase blocks entry into mitosis in the presence of damaged DNA. This checkpoint is activated by signalling from the ATM (ataxia-telangiectasia-mutated) and ATR (ATM and Rad3-related) kinases through phosphorylation of downstream targets such as CHK1 (ref. 1 ). The critical function of the checkpoint is the inhibition of cyclin-dependent kinase (CDK) activity that drives the G2-to-M cell cycle transition. Once repair is completed, the checkpoint is inactivated and CDK activity is increased to promote cell cycle progression [2] . A number of significant biological findings have increased our understanding of checkpoint activation. However, it is not clear how the checkpoint maintenance phase is regulated, particularly following the first wave of kinase-dependent G2 checkpoint control. The p53 tumour suppressor plays a major role in late stages of checkpoint maintenance [3] , [4] , which also suppresses CDK activities. Notably, there is a major gap in our understanding of checkpoint maintenance control during the intermediate phase of the checkpoint following the kinase-driven stage and before the p53-regulated late stage. It is crucial to understand how this phase of the checkpoint is mediated, because poor checkpoint maintenance can result in unscheduled mitotic entry and proliferation of cells with a damaged genome. An emerging factor in genome maintenance is cyclin F, which is not a bona fide CDK-activating cyclin, but an F-box protein belonging to the Skp1-Cullin-F-box (SCF) ubiquitin ligase type family [5] . Previously, NUSAP1 and RRM2 have been described as cyclin F substrates [6] , [7] . Furthermore, cyclin F was described to regulate mitotic progression through control of centrosomal function by degrading CP110 (ref. 8 ). However, a role in checkpoint control has not yet been reported. The oncoprotein B-Myb is a key regulator in the switch between transcriptional repression and activation of a large number of genes including PLK1 , Aurora A , Cyclin A and Cyclin B1/2 during cell cycle progression through the G2 phase [9] , [10] , [11] . B-Myb is part of the transcriptionally activating Myb–MuvB complex, which binds to the CHR promoter elements thereby replacing the DREAM repressor complex [9] . Interestingly, binding of B-Myb was observed in promoters of many genes controlling the transition from G2 to M phase, and contact to promoter regions appeared to depend on the CHR element, but not on Myb-binding sites [11] . Consistently, B-Myb is thought to be required for the cell cycle recovery from the DNA damage-induced G2 checkpoint [12] . Here, we show that cyclin F plays an important role in DNA damage checkpoint control when cells are exposed to ionizing radiation (IR). Cyclin F promotes checkpoint control in the G2 phase by suppression of the B-Myb-driven transcriptional programme that mediates accumulation of mitosis-promoting factors. Cyclin F interacts with B-Myb to suppress cyclin A-mediated phosphorylation of B-Myb, thereby preventing B-Myb activation. In conclusion, we have uncovered a regulatory mechanism linking the F-box protein cyclin F with suppression of the B-Myb/cyclin A pathway to promote the DNA damage checkpoint response in the G2 phase of the cell cycle. Ubiquitome screen identifies a checkpoint role for cyclin F Genes related to ubiquitylation processes play important roles in cell proliferation control [13] . To identify possible new connections between genes involved in ubiquitylation and checkpoint pathways, we searched for new G2 checkpoint regulators following IR with a high-throughput small interfering RNA (siRNA) screen ( Fig. 1a ). The siRNA library was custom-made and it targets 559 genes involved in ubiquitylation pathways. The screen was performed in the human osteosarcoma cell line U2OS expressing an inducible dominant-negative p53 (U2OS-p53dneg) [14] . p53 is not required for the checkpoint at the time points analysed here [3] , and p53 ablation allows for more uniform screening conditions since a number of library siRNAs can induce p53 to disturb cell cycle progression even in the absence of IR. In case the G2 checkpoint is abrogated upon siRNA transfection, cells overcome the IR-induced G2 checkpoint and progress into mitosis where they can be detected by staining for the mitotic marker, Histone H3S10-p. This screen, previously developed in our laboratory, already led to the discovery of a new role for BRCA2 and PALB2 in checkpoint signalling [14] . Data from the screen were statistically analysed to identify candidate genes [15] ( Supplementary Fig. 1a–c ). 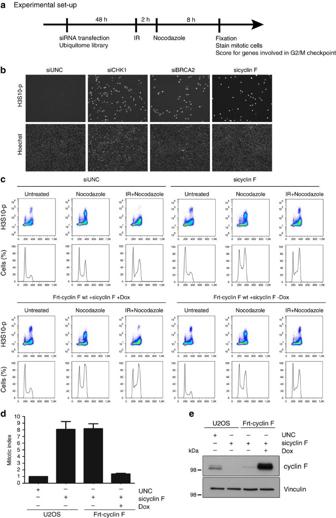Figure 1: Ubiquitome library screen identifies a role for cyclin F in the IR-induced G2 checkpoint. (a) Schematic overview of the automated DNA damage checkpoint siRNA screen with an ubiquitome library. p53 dominant-negative U2OS (p53 dneg U2OS) cells were reverse transfected, incubated for 2 days, irradiated with 6 Gy of IR and 2 h later Nocodazole (Noco) was added for 8 h. The cells were fixed and stained with anti-H3S10-p antibody and Hoechst and analysed for genes regulating the G2 checkpoint. (b) 384-well-plate images from the screen showing control (UNC), CHK1, BRCA2 and cyclin F-depleted cells. (c) U2OS or Frt-Cyclin F siRNA-resistant cells were depleted for control (UNC) or cyclin F. Twenty-four hours after transfection, doxycyclin was added where indicated to express the siRNA-resistant version of cyclin F. After another 24 h, cells were irradiated with 6 Gy of IR, left for 2 h, treated with Nocodazole for 7 h and harvested for flow cytometry. (d) Quantitative analysis of the experiment described inc. Mitotic index is calculated as IR-Noco/Noco relative to the control (UNC). s.e.m. is calculated from three independent experiments. (e) Immunoblot showing cyclin F depletion and overexpression corresponding to the samples incandd. Figure 1: Ubiquitome library screen identifies a role for cyclin F in the IR-induced G2 checkpoint. ( a ) Schematic overview of the automated DNA damage checkpoint siRNA screen with an ubiquitome library. p53 dominant-negative U2OS (p53 dneg U2OS) cells were reverse transfected, incubated for 2 days, irradiated with 6 Gy of IR and 2 h later Nocodazole (Noco) was added for 8 h. The cells were fixed and stained with anti-H3S10-p antibody and Hoechst and analysed for genes regulating the G2 checkpoint. ( b ) 384-well-plate images from the screen showing control (UNC), CHK1, BRCA2 and cyclin F-depleted cells. ( c ) U2OS or Frt-Cyclin F siRNA-resistant cells were depleted for control (UNC) or cyclin F. Twenty-four hours after transfection, doxycyclin was added where indicated to express the siRNA-resistant version of cyclin F. After another 24 h, cells were irradiated with 6 Gy of IR, left for 2 h, treated with Nocodazole for 7 h and harvested for flow cytometry. ( d ) Quantitative analysis of the experiment described in c . Mitotic index is calculated as IR-Noco/Noco relative to the control (UNC). s.e.m. is calculated from three independent experiments. ( e ) Immunoblot showing cyclin F depletion and overexpression corresponding to the samples in c and d . Full size image The ubiquitome library screen revealed several new screen hits, and among these was cyclin F (CCNF) as a candidate regulator of the G2 checkpoint ( Fig. 1b ; Supplementary Fig. 1d ). A role for cyclin F in checkpoint control has not yet been reported. To confirm the findings from the screen, we transfected cells with two siRNAs targeting cyclin F. Cells were then treated with IR and Nocodazole, a mitotic spindle poison, which traps checkpoint-deficient cells entering mitosis. In agreement with the screen finding, cyclin F-depleted cells displayed marked abrogation of the G2 checkpoint in U2OS cells ( Supplementary Fig. 1f ) and human fibroblasts (TIG-3 cells, Supplementary Fig. 1g ). As a further means of validation, we generated a cell line expressing a doxycycline-inducible, siRNA-resistant version of cyclin F (Frt-Cyclin F). Transfection of this cell line with cyclin F siRNA resulted in abrogation of the IR-induced checkpoint. However, the checkpoint was rescued upon induced expression of cyclin F ( Fig. 1c–e ; Supplementary Fig. 1e ). This result strongly suggests that cyclin F is important for the IR-induced G2 checkpoint and that the checkpoint abrogation was directly caused by cyclin F depletion and not by off-target effects. Expression of the cyclin F transgene or cyclin F depletion in the absence of DNA damage did not markedly affect the cell cycle and, importantly, cyclin F-depleted cells were not prone to accumulate in mitosis, thereby ruling out a false-positive screen hit ( Fig. 1c ; Supplementary Fig. 1e ). Cyclin F maintains the IR-induced G2 checkpoint The G2 checkpoint consists of several phases and is initially dependent on ATM and CHK1 (refs 16 , 17 , 18 , 19 ). We investigated whether this initial part of the checkpoint requires cyclin F by harvesting cyclin F-depleted cells for flow cytometry at early time points after IR. This analysis revealed that the IR-induced G2 checkpoint was activated in cyclin F-depleted cells, as seen by the low mitotic index at early time points of 2 and 4 h after IR ( Fig. 2a ). However, cyclin F-depleted cells overcame the G2 arrest at later time points of 6 h after IR and onwards, indicating that cyclin F promotes maintenance rather than activation of the checkpoint ( Fig. 2a ). It was also possible that cyclin F-depleted cells were particularly efficient in DNA repair, for example, via the fast non-homologous end joining pathway, which would allow for rapid cell cycle recovery. We stained cells for γH2AX, an established DNA damage marker [20] , to investigate whether cells entering mitosis contained unrepaired DNA damage. Flow cytometry and immunofluorescence analysis revealed that cyclin F-depleted cells that were captured in mitosis after IR and Nocodazole treatment contained similar levels of γH2AX staining as CHK1-depleted cells receiving the same treatment ( Fig. 2b ; Supplementary Fig. 2a ). On the basis of this analysis, it appears that cells depleted for cyclin F enter mitosis with damaged DNA. Altogether, these data suggest that cyclin F-depleted cells are able to activate the G2 checkpoint, but their checkpoint maintenance is compromised. 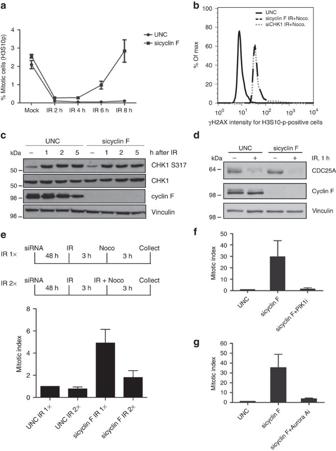Figure 2: Cyclin F is required for maintenance of the IR-induced G2 checkpoint. (a) Checkpoint activation/maintenance in p53 dneg U2OS cells. Cells were depleted with control (UNC) or cyclin F siRNA for 48 h, irradiated with 6 Gy of IR and harvested for flow cytometry at 0, 2, 4, 6 and 8 h after IR, as indicated. Nocodazole was added at the 2-h time point. s.e.m. is calculated from three independent experiments. (b) Cells were treated as inFig. 1aincluding CHK1 depletion as a positive control, and mitotic cells were gated for γH2AX-positive cells. Control contains all mitotic cells in control (UNC)-depleted sample. (c) Checkpoint signalling after IR treatment was monitored in p53 dneg U2OS cells transfected with control (UNC) or cyclin F siRNA for 48 h and immunoblotted for phospho-CHK1-S317 and CHK1 antibodies to assess checkpoint activation. (d) U2OS cells transfected with control (UNC) or cyclin F siRNA for 48 h were treated with IR (6 Gy) followed by 1 h of recovery. CDC25A, cyclin F and vinculin were detected by immunoblotting. (e) Checkpoint recovery in cyclin F-depleted cells is blocked by a delayed subsequent dose of IR. U2OS cells were transfected with control (UNC) or siCyclin F, 48 h following transfection cells were exposed to 6 Gy IR with Nocodazole added 3 h later (IR 1 × ). For repeated IR exposure (IR 2 × ), cells were exposed to a second dosage of IR (6 Gy) 3 h following the initial exposure and Nocodazole added at this time. Irradiated and control cells were incubated with Nocodazole for 3 h and collected for flow cytometry analysis and mitotic index calculation as above. Error bars represent s.e.m. (n=3). (f,g) Flow cytometric analysis of p53 dneg U2OS cells transfected with UNC or cyclin F siRNA. Forty-eight hours after transfection, cells were irradiated with 6 Gy and treated with Nocodazole 2 h later for 7 h. The PLK1 inhibitor (Plk1i: BI2536) or Aurora A inhibitor (Aurora Ai: MLN8054) was added 2 h after IR. The mitotic index was analysed by flow cytometry using anti-H3S10-p. Error bars indicate s.e.m. (n=3). Figure 2: Cyclin F is required for maintenance of the IR-induced G2 checkpoint. ( a ) Checkpoint activation/maintenance in p53 dneg U2OS cells. Cells were depleted with control (UNC) or cyclin F siRNA for 48 h, irradiated with 6 Gy of IR and harvested for flow cytometry at 0, 2, 4, 6 and 8 h after IR, as indicated. Nocodazole was added at the 2-h time point. s.e.m. is calculated from three independent experiments. ( b ) Cells were treated as in Fig. 1a including CHK1 depletion as a positive control, and mitotic cells were gated for γH2AX-positive cells. Control contains all mitotic cells in control (UNC)-depleted sample. ( c ) Checkpoint signalling after IR treatment was monitored in p53 dneg U2OS cells transfected with control (UNC) or cyclin F siRNA for 48 h and immunoblotted for phospho-CHK1-S317 and CHK1 antibodies to assess checkpoint activation. ( d ) U2OS cells transfected with control (UNC) or cyclin F siRNA for 48 h were treated with IR (6 Gy) followed by 1 h of recovery. CDC25A, cyclin F and vinculin were detected by immunoblotting. ( e ) Checkpoint recovery in cyclin F-depleted cells is blocked by a delayed subsequent dose of IR. U2OS cells were transfected with control (UNC) or siCyclin F, 48 h following transfection cells were exposed to 6 Gy IR with Nocodazole added 3 h later (IR 1 × ). For repeated IR exposure (IR 2 × ), cells were exposed to a second dosage of IR (6 Gy) 3 h following the initial exposure and Nocodazole added at this time. Irradiated and control cells were incubated with Nocodazole for 3 h and collected for flow cytometry analysis and mitotic index calculation as above. Error bars represent s.e.m. ( n =3). ( f , g ) Flow cytometric analysis of p53 dneg U2OS cells transfected with UNC or cyclin F siRNA. Forty-eight hours after transfection, cells were irradiated with 6 Gy and treated with Nocodazole 2 h later for 7 h. The PLK1 inhibitor (Plk1i: BI2536) or Aurora A inhibitor (Aurora Ai: MLN8054) was added 2 h after IR. The mitotic index was analysed by flow cytometry using anti-H3S10-p. Error bars indicate s.e.m. ( n =3). Full size image To further investigate the checkpoint activation phase in cells depleted for cyclin F, we analysed key checkpoint markers by western blotting. We depleted cyclin F in the presence or absence of IR and immunoblotted for the phosphorylated version of the checkpoint protein CHK1. This experiment revealed that CHK1 was activated upon IR in both control and cyclin F-depleted cells ( Fig. 2c ), resulting in downregulation of CDC25A protein levels ( Fig. 2d ), which is essential for G2 checkpoint activation [21] . Since checkpoint activation occurred independently of cyclin F, we reasoned that adding continuous DNA damage or a second delayed dose of IR would lead to prolonged checkpoint control. To test this, we irradiated cells twice with a 3-h delay to mediate checkpoint reactivation at the 3-h time point. This second IR dose led to a marked checkpoint arrest after cyclin F depletion ( Fig. 2e ). Furthermore, extended presence of the potent radiomimetic Neocarzinostatin led to continuous DNA damage induction and extended G2 checkpoint control even in cyclin F-depleted cells. In contrast, cyclin F-depleted cells were unable to maintain the checkpoint when the radiomimetic was added for a brief period and subsequently removed ( Supplementary Fig. 2b ). These results suggest that cyclin F promotes checkpoint maintenance only after the checkpoint activating kinase-mediated phase has declined. Next, we investigated whether cyclin F operates prior to p53 as indicated by our data from U2OS cells with disabled p53 ( Fig. 1b ). We depleted cyclin F in the isogenic HCT116 cell lines with and without p53 and harvested cells at 8 h post IR, which is during the period where p53 has little impact on the G2 checkpoint. We found that cyclin F plays an important checkpoint role in the presence and absence of p53 ( Supplementary Fig. 2c ), further supporting our notion that cyclin F operates prior to p53 during G2 checkpoint control. Cells exit the checkpoint in an active recovery process where they re-enter the cell cycle upon completion of DNA damage repair. The Aurora A/BORA/PLK1 pathway has emerged as an important positive regulator in facilitating recovery from the G2 checkpoint [22] . PLK1 is inactivated in response to IR by suppression of its T210 phosphorylation [23] . We observed an initial reduction (at 3 h post IR) in PLK1-T210 phosphorylation following cyclin F depletion. However, we found that PLK1 phosphorylation reappeared at later time points after IR in the absence of cyclin F ( Supplementary Fig. 2d ), which is in agreement with our notion that cyclin F regulates G2 checkpoint maintenance. Interestingly, the reintroduction of exogenous cyclin F in cyclin F-depleted cells had a marked impact on PLK1 phosphorylation, since the level of PLK1-T210p remained low throughout the checkpoint similar to control-depleted cells ( Supplementary Fig. 2d ), further supporting a role for cyclin F in checkpoint maintenance. Next, we investigated whether PLK1 or Aurora A inhibition could repress the checkpoint defect observed after cyclin F depletion. We found that co-inhibition of the two proteins (cyclin F/PLK1 and cyclin F/Aurora A) reverted the checkpoint abrogation phenotype observed with cyclin F depletion alone ( Fig. 2f,g ). Collectively, these data suggest that cyclin F promotes G2 checkpoint maintenance by preventing premature checkpoint recovery. Cyclin F regulates the transcriptional activity of B-Myb Due to the known function of cyclin F in promoting the ubiquitylation of target substrates [6] , [7] , [8] , we speculated whether cyclin F could target PLK1 or Aurora A for proteasomal degradation. Indeed, we observed elevated PLK1 and Aurora A protein levels in cells depleted for cyclin F compared with control cells in untreated as well as IR-treated cells ( Supplementary Fig. 3a ). An even more pronounced effect was detected in G2-synchronized cells following IR treatment ( Fig. 3a ). However, the turnover of PLK1 and Aurora A proteins was not affected in cyclin F-depleted cells ( Supplementary Fig. 3b ). In contrast, cyclin F appeared to control messenger RNA (mRNA) levels of PLK1 and Aurora A, as well as the mRNA levels of cyclin A2 and cyclin B2 upon IR treatment ( Fig. 3b ). The increased mRNA levels of these genes following cyclin F depletion could be rescued by complementation with exogenous cyclin F ( Fig. 3b ). In accordance with the immunoblot results, the increased mRNA levels of PLK1, Aurora A and cyclin B were especially pronounced upon IR treatment ( Supplementary Fig. 3c ). Furthermore, the promoter activities of the PLK1 and cyclin B2 genes were enhanced by cyclin F depletion ( Supplementary Fig. 3d ). These findings indicate a role for cyclin F in repressing transcription of genes involved in mitotic entry rather than in mediating their proteasomal degradation. 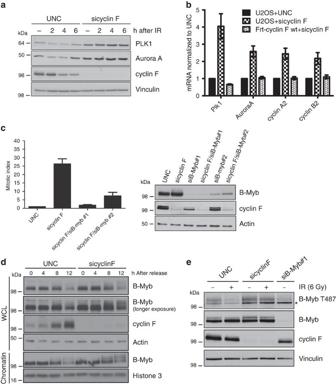Figure 3: Cyclin F is involved in controlling the transcriptional activity of B-Myb. (a) U2OS cells were transfected with control (UNC) or cyclin F siRNA. The cells were synchronized by a double thymidine block and released for 8.5 h, followed by IR treatment (6 Gy). Cells were harvested 0 (−), 2, 4 and 6 h after IR and processed for immunoblotting. (b) U2OS or Frt-Cyclin F siRNA-resistant cells were transfected with UNC or cyclin F siRNA. After 48 h, cells were treated with IR (6 Gy) and harvested 6 h later. RNA was extracted, cDNA generated and relative numbers of transcripts were analysed by quantitative PCR. The expression levels of transcripts were normalized to the housekeeping geneubiquitinin all samples. The values were subsequently normalized to the IR-treated control (UNC transfected) sample. Error bars indicate s.e.m. (n=3). (c) Left panel: U2OS p53 dneg cells were transfected with control (UNC) or cyclin F siRNA with or without B-Myb#1/#2 siRNA. After 48 h, cells were irradiated (6 Gy), 2 h later treated with Nocodazole for 7 h and harvested for flow cytometry to detect mitotic cells using anti-H3S10-p. Error bars indicate s.e.m. (n=3). Right panel: immunoblot of U2OS p53 dneg cells depleted for cyclin F and/or B-Myb#1/#2 for 2 days. (d) U2OS cells were transfected with control (UNC) or cyclin F siRNA. The cells were synchronized by a double thymidine block and released for the indicated time points. The whole-cell lysates and chromatin fractions were analysed by immunoblotting. (e) U2OS cells were transfected with control (UNC), cyclin F or B-Myb siRNA. The cells were synchronized by a double thymidine block, released for 8 h and left untreated or treated with IR (6 Gy) followed by harvesting 3 h later. The whole-cell lysates were analysed by immunoblotting with phospho-B-Myb-T487, B-Myb, cyclin F and vinculin antibodies. The asterisk denotes an unspecific band. Figure 3: Cyclin F is involved in controlling the transcriptional activity of B-Myb. ( a ) U2OS cells were transfected with control (UNC) or cyclin F siRNA. The cells were synchronized by a double thymidine block and released for 8.5 h, followed by IR treatment (6 Gy). Cells were harvested 0 (−), 2, 4 and 6 h after IR and processed for immunoblotting. ( b ) U2OS or Frt-Cyclin F siRNA-resistant cells were transfected with UNC or cyclin F siRNA. After 48 h, cells were treated with IR (6 Gy) and harvested 6 h later. RNA was extracted, cDNA generated and relative numbers of transcripts were analysed by quantitative PCR. The expression levels of transcripts were normalized to the housekeeping gene ubiquitin in all samples. The values were subsequently normalized to the IR-treated control (UNC transfected) sample. Error bars indicate s.e.m. ( n =3). ( c ) Left panel: U2OS p53 dneg cells were transfected with control (UNC) or cyclin F siRNA with or without B-Myb#1/#2 siRNA. After 48 h, cells were irradiated (6 Gy), 2 h later treated with Nocodazole for 7 h and harvested for flow cytometry to detect mitotic cells using anti-H3S10-p. Error bars indicate s.e.m. ( n =3). Right panel: immunoblot of U2OS p53 dneg cells depleted for cyclin F and/or B-Myb#1/#2 for 2 days. ( d ) U2OS cells were transfected with control (UNC) or cyclin F siRNA. The cells were synchronized by a double thymidine block and released for the indicated time points. The whole-cell lysates and chromatin fractions were analysed by immunoblotting. ( e ) U2OS cells were transfected with control (UNC), cyclin F or B-Myb siRNA. The cells were synchronized by a double thymidine block, released for 8 h and left untreated or treated with IR (6 Gy) followed by harvesting 3 h later. The whole-cell lysates were analysed by immunoblotting with phospho-B-Myb-T487, B-Myb, cyclin F and vinculin antibodies. The asterisk denotes an unspecific band. Full size image The oncoprotein B-Myb is an important transcriptional activator of genes that promote mitotic entry, such as PLK1 , Cyclin A and Cyclin B [9] , [10] . This activity of B-Myb is thought to explain how it promotes recovery from the DNA damage-induced G2 checkpoint [12] . To investigate whether cyclin F and B-Myb are functionally linked in regulating the G2/M checkpoint, we co-depleted B-Myb and cyclin F and treated the cells with IR to induce DNA damage. Subsequent analysis by flow cytometry revealed that the G2 checkpoint was maintained suggesting that B-Myb is required for mitotic entry when cyclin F is depleted ( Fig. 3c ; Supplementary Fig. 3e ). Next, we wanted to test whether cyclin F regulates B-Myb protein levels or its transcriptional activity. Cyclin F depletion affected neither B-Myb protein stability nor mRNA levels ( Supplementary Fig. 3f ; Fig. 4d ). B-Myb activity is regulated by post-translational modifications and protein–protein interactions [24] . In S and G2 phases, B-Myb is activated by cyclin A–CDK2-mediated phosphorylation that releases B-Myb from repressors [25] , [26] , [27] , [28] , [29] . We observed an increase in B-Myb phosphorylation in cyclin F-depleted cells that could be reversed by phosphatase treatment ( Supplementary Fig. 3g ), indicating a potential role for cyclin F in regulating B-Myb activity. Chromatin-bound B-Myb appeared to be strongly hyperphosphorylated in G2 and M phases in cells depleted for cyclin F compared with control-depleted cells ( Fig. 3d ). In cells transfected with control siRNA (UNC), B-Myb phosphorylation decreased upon IR treatment ( Fig. 3e ). Remarkably, cyclin F depletion not only increased B-Myb phosphorylation in untreated cells, but also maintained the B-Myb phosphorylation upon IR treatment, as shown by the use of a B-Myb phospho-specific antibody recognizing T487 phosphorylated by cyclin A–CDK2 (ref. 25 ) ( Fig. 3e ). These findings suggest a role for cyclin F in restricting B-Myb activation especially in response to DNA damage. 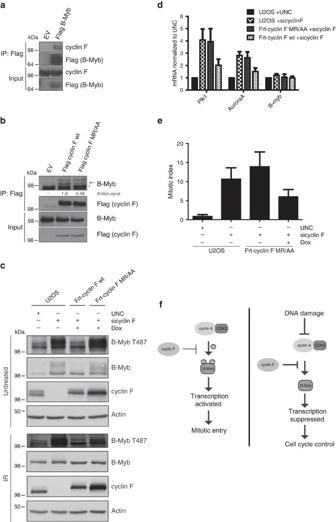Figure 4: Cyclin F regulates B-Myb activity via its hydrophobic patch motif. (a) HEK293 cells were transfected with empty vector (EV) or mouse FLAG B-Myb expression plasmids, and subjected to FLAG-immunoprecipitation followed by immunoblotting with anti-cyclin F and anti-FLAG antibodies. (b) HEK293 cells were transfected with EV, FLAG Cyclin F wt or cyclin F hydrophobic patch mutant (MR/AA) expression plasmids, and subjected to immunoprecipitation with FLAG beads. Lysates and immunoprecipitates were analysed by immunoblotting. The arrow indicates the co-precipitated endogenous B-Myb, and numbers below the panels represent quantification of the B-Myb band. The asterisk denotes an unspecific band. (c) U2OS cells or cells expressing siRNA-resistant Frt-Cyclin F wild-type (wt) or MR/AA mutant were transfected with indicated siRNAs. Cells were then synchronized with a double thymidine block and released for 8 h followed by IR as indicated (6 Gy). After 3 h, cells were harvested and analysed by immunoblotting with phospho-B-Myb-T487, B-Myb, cyclin F and actin antibodies. (d) U2OS cells, Frt-cyclin F wild-type or MR/AA mutant siRNA-resistant cells were transfected with siRNA. After 48 h, cells were treated with IR (6 Gy) and harvested 3 h later. RNA was extracted, cDNA generated and relative numbers of transcripts were analysed by quantitative PCR. Values were normalized to the IR-treated control (UNC transfected) sample. Error bars indicate s.e.m. (n=5). (e) U2OS or Frt-Cyclin F MR/AA mutant siRNA-resistant cells were depleted for 48 h as indicated. Twenty-four hours after transfection, doxycycline was added to induce the siRNA-resistant version of cyclin F. After another 24 h, cells were irradiated with 6 Gy of IR, left for 2 h, treated with Nocodazole for 7 h and harvested for flow cytometry. Error bars indicate s.e.m. (n=3). (f) Cyclin F regulates B-Myb transcriptional activity to guard against unscheduled mitotic entry in the presence of unrepaired DNA lesions. In the absence of damage, cyclin F-mediated control of B-Myb has little impact on cell proliferation (left side of the figure). However, when cells are challenged with IR, cyclin F suppresses the activating CDK–cyclin A-mediated phosphorylation of B-Myb and thereby the transcriptional programme that promotes progression through the G2 phase into mitosis (right side of the figure). Figure 4: Cyclin F regulates B-Myb activity via its hydrophobic patch motif. ( a ) HEK293 cells were transfected with empty vector (EV) or mouse FLAG B-Myb expression plasmids, and subjected to FLAG-immunoprecipitation followed by immunoblotting with anti-cyclin F and anti-FLAG antibodies. ( b ) HEK293 cells were transfected with EV, FLAG Cyclin F wt or cyclin F hydrophobic patch mutant (MR/AA) expression plasmids, and subjected to immunoprecipitation with FLAG beads. Lysates and immunoprecipitates were analysed by immunoblotting. The arrow indicates the co-precipitated endogenous B-Myb, and numbers below the panels represent quantification of the B-Myb band. The asterisk denotes an unspecific band. ( c ) U2OS cells or cells expressing siRNA-resistant Frt-Cyclin F wild-type (wt) or MR/AA mutant were transfected with indicated siRNAs. Cells were then synchronized with a double thymidine block and released for 8 h followed by IR as indicated (6 Gy). After 3 h, cells were harvested and analysed by immunoblotting with phospho-B-Myb-T487, B-Myb, cyclin F and actin antibodies. ( d ) U2OS cells, Frt-cyclin F wild-type or MR/AA mutant siRNA-resistant cells were transfected with siRNA. After 48 h, cells were treated with IR (6 Gy) and harvested 3 h later. RNA was extracted, cDNA generated and relative numbers of transcripts were analysed by quantitative PCR. Values were normalized to the IR-treated control (UNC transfected) sample. Error bars indicate s.e.m. ( n =5). ( e ) U2OS or Frt-Cyclin F MR/AA mutant siRNA-resistant cells were depleted for 48 h as indicated. Twenty-four hours after transfection, doxycycline was added to induce the siRNA-resistant version of cyclin F. After another 24 h, cells were irradiated with 6 Gy of IR, left for 2 h, treated with Nocodazole for 7 h and harvested for flow cytometry. Error bars indicate s.e.m. ( n =3). ( f ) Cyclin F regulates B-Myb transcriptional activity to guard against unscheduled mitotic entry in the presence of unrepaired DNA lesions. In the absence of damage, cyclin F-mediated control of B-Myb has little impact on cell proliferation (left side of the figure). However, when cells are challenged with IR, cyclin F suppresses the activating CDK–cyclin A-mediated phosphorylation of B-Myb and thereby the transcriptional programme that promotes progression through the G2 phase into mitosis (right side of the figure). Full size image Cyclin F regulates B-Myb activity via the cyclin box domain Cyclin F does not bind to CDKs but has a cyclin box domain, which contains a hydrophobic patch motif [8] , [30] , [31] . In cyclin F, this hydrophobic patch with the amino-acid sequence MRYIL (Met-Arg-Tyr-Ile-Leu) associates with the Cy-motif (arginine-X-leucine) in its substrates [6] , [8] . To further investigate the interplay between cyclin F and B-Myb, we performed immunoprecipitation (IP) experiments to probe for an interaction between the two proteins, and we were able to co-immunoprecipitate cyclin F with Flag-tagged B-Myb ( Fig. 4a ). We then co-incubated purified recombinant glutathione S-transferase (GST)-tagged cyclin F and in vitro translated B-Myb. B-Myb was detected by immunoblotting following GST pull-down, suggesting that cyclin F and B-Myb can directly interact ( Supplementary Fig. 4a ). Cyclin F contains a number of protein-interacting domains, and we generated truncated versions to further characterize the interaction with B-Myb. Subsequent immunoprecitation of B-Myb revealed that cyclin F associates with B-Myb via the central cyclin box domain ( Supplementary Fig. 4b ). Consequently, we investigated whether the interaction between cyclin F and B-Myb is dependent on the hydrophobic patch in cyclin F. Indeed, less B-Myb was co-immunoprecipitated with cyclin F containing a mutation in the hydrophobic patch (MR/AA) compared with cyclin F wild type (wt) ( Fig. 4b ). Cyclin A may also bind to B-Myb via its hydrophobic patch motif subsequently leading to CDK-dependent B-Myb phosphorylation and activation [25] , [26] , [27] , [28] , [29] , [32] . Therefore, we reasoned that cyclin F could interfere with cyclin A–CDK2-mediated phosphorylation of B-Myb, thereby suppressing the cell cycle-promoting activity of B-Myb. In accordance with this notion, co-depletion of cyclin F and cyclin A reverted the checkpoint abrogation phenotype induced by cyclin F depletion alone ( Supplementary Fig. 4c ). Moreover, the kinase activity associated with cyclin A was not affected by cyclin F depletion, further supporting the idea that cyclin F interferes with cyclin A-dependent activation of B-Myb rather than affecting cyclin A kinase activity directly ( Supplementary Fig. 4d ). Having established a role for the hydrophobic patch in cyclin F for B-Myb interaction, we investigated the role of this motif in B-Myb transcriptional control and the G2 checkpoint. Importantly, complementation with siRNA-resistant wt cyclin F rescued the increase in B-Myb phosphorylation that was observed in cyclin F-depleted cells, whereas the expression of the MR/AA mutant cyclin F led to a persistent increase in B-Myb phosphorylation compared with control-depleted cells ( Fig. 4c ). This result suggests that the hydrophobic patch in cyclin F plays an important role in the control of B-Myb activity, and that the MR/AA mutant is a loss-of-function version. In line with this, complementation with the MR/AA mutant allowed elevated mRNA levels of PLK1 and Aurora A ( Fig. 4d ). Furthermore, unlike the wt version ( Fig. 1c,d ), the MR/AA mutant could not complement the checkpoint function of cyclin F ( Fig. 4e ). Taken together, our data uncover the importance of the cyclin box domain in cyclin F in mediating the regulation of B-Myb activity. In summary, our results show that cyclin F suppresses B-Myb activity to maintain the G2 checkpoint following IR. Furthermore, our data support a model where combined control of B-Myb is required to avoid unscheduled mitotic entry in the presence of DNA damage ( Fig. 4f ). In undamaged cells, our data suggest that cyclin F-mediated control of B-Myb has little impact on transcriptional activation and hence cell proliferation, although the phosphorylation of B-Myb is still affected by the presence of cyclin F. However, when cells are challenged with DNA damage such as IR, we propose that B-Myb is initially suppressed by two pathways impinging on the cyclin A–CDK-mediated B-Myb activation. First, the G2 phase action of cyclin F serves to limit B-Myb phosphorylation and thereby promote the ability to target the B-Myb pathway. This regulatory action is subsequently supported by the DNA damage checkpoint-mediated inhibition of cyclin A–CDK2 kinase activity, which is achieved through inhibition of CDC25 phosphatase activity. In this way, the B-Myb-driven transcriptional programme that promotes progression through the G2 phase into mitosis is suppressed until the DNA damage is repaired. In addition to the functional data linking B-Myb and cyclin F, it is also evident that cyclin F can directly interact with B-Myb. This interaction appears to be mediated via the cyclin box domain of cyclin F, which directs cyclin F protein substrates for ubiquitiylation and subsequent degradation [5] . Notably, B-Myb harbours multiple cyclin-binding sites (Cy-motifs) dispersed throughout the entire sequence, and consistent with this, we were unable to map a single B-Myb region required for the interaction with cyclin F. On the basis of this, we now propose that B-Myb makes multiple independent Cy-motif-based contacts with cyclin F. Intriguingly, we have so far not identified a role for cyclin F-mediated protein turnover in checkpoint control, and although protein degradation remains a contributing possibility, we favour alternative mechanistic explanations for the role of cyclin F. First, we propose that cyclin F may directly compete with cyclin A for binding to B-Myb, thereby suppressing B-Myb phosphorylation and activation. Furthermore, cyclin F may actively support B-Myb dephosphorylation, for example, by recruiting a phosphatase to the complex with B-Myb. Clearly, the mechanism by which cyclin F regulates B-Myb remains to be precisely determined, which is an important line of future research. Importantly, this cyclin F pathway operates prior to the p53-mediated response to DNA damage, as p53 initially has a modest role in the G2 checkpoint for the first 12 h after DNA damage [3] , [4] . The p53-mediated checkpoint control is exerted later primarily by indirect repression of transcription of many G2–M-controlling genes [33] . Interestingly, it was recently shown by a meta-analysis of genome-wide expression data that the MYBL2 gene encoding B-Myb is indirectly downregulated by p53 contributing to G2 checkpoint control [33] . Taken together, the cyclin F-mediated regulatory mechanism adds a new layer of cell cycle control in the early response to DNA damage. We therefore propose that the transcriptional suppression mediated by cyclin F serves as an important temporal safeguard maintaining repression of target genes until the p53 response eventually contributes through mechanisms such as the p53-p21-DREAM-CDE/CHR pathway [34] , [35] . Very interestingly, cyclin F has been shown to be reduced in certain cancer types [36] , whereas B-Myb is overexpressed in several types of cancers [37] . It has been reported that low cyclin F levels correlate with poor differentiation and unfavourable prognosis in hepatocellular carcinoma [36] . It is therefore possible that cyclin F plays a relevant role in cancer development by preventing unscheduled cell proliferation and genomic instability through the suppression of B-Myb. Cells and reagents The human osteosarcoma cell line (U2OS) and U2OS cells expressing a dominant-negative version of p53 (p53dneg) in a tet-off system were grown in Dulbecco’s modified Eagle’s medium with 10% fetal bovine serum (FBS) (containing doxycycline, 1 ng ml −1 , for the U2OS-p53dneg cells). To express the dominant-negative version of p53 (p53dneg), cells were washed two times in PBS and grown in medium without doxycycline. Furthermore, human-telomerized fibroblasts (TIG-3) and human embryonic kidney 293 cells (HEK293) were grown in Dulbecco’s modified Eagle’s medium with 10% FBS. HCT116 and HCT116 P53 knockout cells as described by Bunz et al . [3] were cultured in McCoy’s 5A media containing 10% FBS. Stable U2OS cell lines expressing the Flag-haemagglutinin (HA)-tagged siRNA-resistant versions of cyclin F wt (Frt-Cyclin F wt) and cyclin F mutated in the hydrophobic patch motif (MR-AA; Frt-Cyclin F MR/AA) were established. For that, cyclin F wt complementary DNA (cDNA) was cloned into pcDNA5-Frt-TO vector (Invitrogen). The cyclin F transcript was rendered siRNA resistant towards siRNA-cyclin F#1 by site-directed mutagenesis with the primers FW 5′- CTGGGAAAGCGACAGGAGAACCGACGTGTCGGATCCTGGGCGATGCCTCT -3′ and RV 5′- AGAGGCATCGCCCAGGATCCGACACGTCGGTTCTCCTGTCGCTTTCCCAG -3′. The PFU-Ultra High-Fidelity Polymerase (Stratagene) was used according to the manufacturer’s protocol. The mutation of the hydrophobic patch MRYIL (amino acid 309–313) in the cyclin domain of cyclin F to AAYIL (MR/AA) was introduced into the siRNA-resistant cyclin F pcDNA5-Frt-TO vector by site-directed mutagenesis. The primers FW 5′- GGGACTCAATGACACAGCGGCGTACATTCTGATCGACTGG -3′ and RV 5′- CCAGTCGATCAGAATGTACGCCGCTGTGTCATTGAGTCCC -3′ were used. The siRNA-resistant cyclin F plasmids were then co-transfected with Flp recombinase (pOG44, Invitrogen) into U2OS-Frt-Trex cells by FuGene (Roche) according to the manufacturer’s protocol, resulting in a cell line expressing FLAG-HA-tagged siRNA-resistant cyclin F (denoted Frt-Cyclin F) in a tet-on system. These cells were grown in Dulbecco’s modified Eagle’s medium with 10% FBS (Tet-system-approved FBS, Clontech). To induce expression of siRNA-resistant cyclin F, doxycycline (1 ng ml −1 ) was added to the medium for ~24 h. The truncated cyclin F expression constructs were generated by PCR using the cyclin F entry vector (pENTR, Invitrogen). The following primers were used: Cyclin F aa 1–271 5′- CACCATGGGGAGCGGCGGCGTGGT -3′ and 5′- TTACTGGTTTGCATTTGCACAGGCTTTGGC -3′, for Cyclin F aa 1–581 5′- CACCATGGGGAGCGGCGGCGTGGT -3′ and 5′- TTAGTCTTCCTGGAGGCTGTTCTCCCGCTT -3′ and for cyclin F aa 264–787 5′- CACCATGAAAGCCTGTGCAAATGCAAACCAG -3′ and 5′- TTACAGCCTCACAAGGCCCA -3′. The green fluorescent protein (GFP)-tagged B-Myb was generated using the human B-Myb entry vector (pCR8/GW/TOPO, Invitrogen). The entry vectors were cloned into the pCMV Minkio HA-FLAG or pCDNA4/TO-GFP expression vectors with the Gateway LR Clonase II enzyme mix (Invitrogen). The reactions were performed according to the manufacturer’s protocol. For siRNA transfections (48 h), Lipofectamine RNAiMAX (Invitrogen) was used according to the manufacturer’s protocol. The oligonucleotide sequences used for knockdown are: cyclin F#1: 5′- GGAGGACAGAUGUGUCAGA [dT][dT], cyclin F#2: 5′- GCGCAGCUGUCUUUAGCCA [dT][dT], CHK1 (#108): 5′- GGGAUAUUAAACCAGAAAA [dT][dT], BRCA2: 5′- CCAACUUUGUCCUUAACUA [dT][dT], B-Myb#1: 5′- GCAGAGGACAGUAUCAACA [dT][dT], B-Myb#2: 5′- GAUCUGGAUGAGCUGCACU [dT][dT], cyclin A: 5′- CCAUUGGUCCCUCUUGAUU [dT][dT] MISSION siRNA Universal Negative Control (UNC, Sigma-Aldrich) was used as a negative control. siCyclin F in figures refers to siCyclin F#1, unless otherwise stated. To transfect HEK293 cells with expression plasmids, the calcium phosphate transfection method was used. Nocodazole, cycloheximide, MG132 and thymidine were used at final concentrations of 100 ng μl −1 , 20 μg ml −1 , 5 μM and 2 mM, respectively (Sigma-Aldrich). Furthermore, PLK1 inhibitor [38] (BI2536, Axon Medchem BV) and Aurora A inhibitor [39] (MLN8054, Selleck) were used at final concentrations of 100 nM and 250 nM, respectively. Neocarzinostatin was obtained from Sigma and used at a concentration of 100 ng ml −1 to induce DNA damage. IR was given using a Faxitron X-ray apparatus calibrated to give 1 Gy gamma irradiation per 2 min. Unless otherwise stated, cells were irradiated with 6 Gy of IR. Cell synchronization U2OS cells (ATCC, number HTB-96) were synchronized via a double thymidine block by treating cells with 2 mM thymidine (Sigma-Aldrich) for 19 h. Cells were then released into fresh media for 9 h followed by a second thymidine block for 15 h. Cells were subsequently released into fresh media and harvested at the indicated time points. Ubiquitome screen The ubiquitome library (Ambion) consisted of siRNAs targeting 559 genes ( Supplementary Data 1 ), with each gene targeted by three different siRNAs spotted individually onto 384-well plates. The ubiquitome screen was performed using an automated liquid-handling station (STAR; Hamilton Robotics). U2OS cells expressing a dominant-negative version of p53 in a tet-off system were reverse-transfected with the siRNAs targeting the human ubiquitome. The transfection was performed as previously described [14] . Briefly, 4 μl siRNA (1 μM) was mixed with 2.5 μl OptiMEM (Invitrogen) in a 384-well plate (Corning). Subsequently, 6.5 μl transfection mix consisting of 6.46 μl OptiMEM+0.04 μl RNAiMAX was added to each well and incubated for 15 min at room temperature to form complexes. To this transfection mix, 2,200 cells in 25 μl medium were added to give a final siRNA concentration of 100 nM. Cells were incubated for 48 h, treated with IR (6 Gy) and Nocodazole (100 ng ml −1 ; Sigma-Aldrich) was added 2 h later for 8 h. The cells were then fixed in 4% formaldehyde, permeabilized in 0.25% Triton X-100/PBS and stained with H3S10-p antibody (Millipore) to be visualized by Alexa Fluor 594 secondary antibody. To the secondary antibody, Hoechst (bisBenzimide H 33342; Sigma-Aldrich) was added to stain the nuclei. Cells were left at 4 °C in PBS before imaging, which was performed on an IN Cell Analyzer 1,000 (GE Healthcare). Ten images per well were acquired using the × 20 objective and ~2,000 cells per well were analysed using the IN Cell Analyzer Workstation 3.5 software (GE Healthcare). Statistical analysis The data obtained from the screen was submitted to a redundant siRNA activity analysis that models the probability of a gene ‘hit’ based on the collective activities of multiple siRNAs per gene [15] . Using this method, the siRNAs were ranked according to their score. Then a P value was assigned to each gene and this value indicated the likelihood of observing a high-scoring gene by chance. The P values were calculated based on the iterative hypergeometric distribution [15] . In our screen, the redundant siRNA activity analysis was performed based on the percentage of H3S10-p-positive cells. Flow cytometry To prepare cells for flow cytometry, cells were fixed in 70% ethanol. The cells were stained with rabbit-anti-phospho-H3S10 antibody (1:200, Millipore) and mouse-anti-γH2AX antibody (1:500, Millipore) for 1 h followed by 1-h incubation with Alexa Fluor 488 anti-mouse and 647 anti-rabbit (1:1,000) secondary antibodies. DNA was stained with 0.1 mg ml −1 propidium iodide containing RNase (20 μg ml −1 ) for 30 min at 37 °C. Flow cytometry was performed on a FACS Calibur (BD Biosciences) using CellQuest Pro software (Becton Dickinson). Immunoblotting and antibodies Briefly, cells were snap-frozen and lysed in cold EBC buffer (150 mM NaCl, 50 mM Tris pH 7.4, 1 mM EDTA, 0.5% Igepal) containing protease inhibitors (1% vol/vol aprotinin, 5 μg ml −1 leupeptin, 1 mM phenylmethylsulphonyl fluoride), phosphatase inhibitors (50 mM NaF, β-glycerophosphate) and 1 mM dithiothreitol. The lysates were sonicated 2 × 2 s at 20% (S250, Branson). The proteins were then separated by SDS–polyacrylamide gel electrophoresis (PAGE) and transferred to a nitrocellulose membrane. The membranes were blocked in 5% milk, incubated with primary antibody diluted in 5% milk, washed and incubated with secondary horseradish peroxidase-conjugated antibody (1:10,000; Vector Laboratories) diluted in 5% milk. ECL-mix (Thermo Scientific) was used to visualize proteins, and films were developed using an X-ray machine (Valsoe; Ferrania Technologies). The following primary antibodies were used for immunoblotting: Aurora A (1:4,000; ab1287, Abcam), phospho-B-MyB-T487 (1:500; ab76009, Abcam), Cyclin A (1:500; H-432, sc751, Santa Cruz), Cyclin B1 (1:2,000; GNS1, sc245, Santa Cruz), Cyclin F (1:5,000; C-20, sc952, Santa Cruz), phospho-CHK1-S317 (1:1,500; 2344L, Cell Signaling), CHK1 (1:10,000; DCS-310; described in ref. 40 ), CDC25A (1:200; F-6, sc7389, Santa Cruz), FLAG (1:5,000; M2, 61415, Sigma), GFP (1:1,000; 11814460001, Roche), HA (1:2,000; MMS-101P, Covance), Histone 3 (1:10,000; ab1791, Abcam), p53 (1:100; DO-1), PLK1 (1:1,000; H152, sc5585, Santa Cruz), phospho-PLK1-T210 (1:200; ADI-KAP-CC107-D, Enzo Life Science), Vinculin (1:50,000; V9131, Sigma) and Actin (1:20,000; mAB1501, Chemicon Int.). The B-Myb LX015.1 monoclonal antibody (1:10) was a kind gift from Roger Watson [41] . B-Myb levels in Fig. 4b were quantified relative to the control IP using ImageJ software. Supplementary Fig. 5 contains uncropped scans of the immunoblots. Cellular fractionation This was performed as described previously [42] . In brief, cells were lysed in CSK buffer (0.5% Triton X-100, 10 mM Pipes, pH 6.8, 300 mM sucrose, 100 mM NaCl and 1.5 mM MgCl 2 ). The lysed cells were pelleted by centrifugation at 1,000 g , and supernatant was collected (soluble fraction). The pellet was washed once with CSK buffer, resuspended in 0.2 M HCl and incubated overnight at 4 °C. The supernatant represented the chromatin-enriched fraction. HCl-containing samples were neutralized with Tris buffer (1.5 M, pH 8.8) before SDS–PAGE. Whole-cell extracts were prepared as decribed below (immunoblotting and antibodies). Immunofluorescence Cells were grown on coverslips and treated as indicated in the figure legends. The coverslips were fixed and stained as described previously [42] . Briefly, the coverslips were fixed in 4% formaldehyde following 2 min of pre-extraction in Triton buffer (0.5% Triton X-100 in 20 mM Hepes, pH 7.4, 50 mM NaCl, 3 mM MgCl and 300 mM sucrose), permeabilized in 0.3% Triton X-100/PBS, blocked in 3% bovine serum albumin and incubated with phospho-H2AX-S139 (1:1,000; JBW103, Millipore) and H3S10-p (1:500, Millipore) antibodies, as indicated. Samples were then stained with species-specific Alexa Fluor 488 and/or 594, washed and mounted in Vectashield mounting medium with 4',6-diamidino-2-phenylindole (Vector Laboratories). Immunoprecipitation Extracts for IP were prepared using IP buffer (50 mM Hepes, pH 7.5, 150 mM NaCl, 1 mM EDTA, 2.5 mM EGTA, 10% glycerol and 0.1% Tween) with protease inhibitors. For IP of ectopically expressed proteins, M2 FLAG beads (Sigma-Aldrich) or GFP-Trap beads (ChromoTek) were washed and incubated with the lysate for 2 h at 4 °C on a rotator. The beads were washed five times followed by elution of bound proteins. Kinase assay Cyclin A antibody was coupled to protein A sepharose beads via rotation for 1 h at 4 °C. Anti-rabbit total IgG coupled to protein A sepharose beads served as a control. U2OS cellular extracts for IP were prepared in IP buffer with protease and phosphatase inhibitors. The lysis mixture was incubated on ice for 15 min, sonicated three times with a digital sonicator for 3 s (20%; S250; Branson) and centrifuged for 10 min at 4 °C. After centrifugation, 20 μl of protein A sepharose conjugated with 0.5 μg of antibody was added to 250 μg cell lysate and the mixture was allowed to precipitate for 1.5 h at 4 °C with rotation. The immune complexes were pelleted by gentle centrifugation and washed three times with 1 ml of IP buffer. IP reactions were subsequently washed twice in 1 ml of kinase buffer (50 mM Hepes, pH 7.4, 10 mM MgCl 2 , 1 mM dithiothreitol, protease inhibitors: leupeptin, aprotinin and phenylmethylsulphonyl fluoride and phosphatase inhibitors: NaF and β-glycerophosphate). After the final wash, kinase buffer (50 μl) was temporarily retained to prevent the drying out of beads. A kinase reaction mixture was prepared and added to the IP reactions in a final volume of 25 μl per sample to be assayed: 50 μM ‘cold’ ATP, 2.5 μg Histone H1, 5μCi [γ-32P]-ATP and kinase buffer. Reactions were incubated for 20 min at 30 °C with gentle agitation. Laemmli buffer was added directly to samples, samples were boiled and reactions were resolved on a 15% SDS–PAGE gel. Resolved proteins were transferred to nitrocellulose membrane overnight at 50 mA and exposed membranes were visualized on a Fujifilm Phosphoimager. Immunoblotting was performed for cyclin A and cyclin F, and Ponceau S staining was employed to confirm equal loading of H1 in all samples. Luciferase assay To measure promoter activity with luciferase reporter assays, U2OS cells were plated in 24-well plates (75,000 cells per well) and transfected by lipofection with Fugene 6 (Promega). Cells were cultured overnight, co-transfected with 150 ng of pGL4 promoter reporter plasmids and 25 ng Renilla luciferase control plasmid, collected and assayed as described [9] . In brief, luciferase activity was measured with the dual-luciferase reporter assay system (Promega) following the manufacturer’s recommendations. Relative light units were calculated by normalizing firefly luciferase activity to Renilla luciferase activity. Quantification of mRNA levels by quantitative PCR Quantitative PCR was performed as described previously [42] . In brief, RNA was purified from U2OS cells using the RNeasy kit (Qiagen). cDNA was generated by reverse transcription-PCR (TaqMan; Applied Biosystems) according to the manufacturer’s protocol. Real-time quantitative PCR was performed employing the LightCycler 480 System (Roche Diagnostics) using the Maxima SYBR Green qPCR Master Mix (Fermentas). Ubiquitin mRNA levels were used as a control for normalization. For amplification of the indicated cDNAs, the following primers were used: PLK1: FW 5′- AAAGAGATCCCGGAGGTCCTA -3′, RV 5′- GGCTGCGGTGAATGGATATTTC -3′ Aurora A: FW 5′- TTCAGGACCTGTTAAGGCTACA -3′, RV 5′- ATTTGAAGGACACAAGACCCG -3′ Cyclin A2: FW 5′- CGCTGGCGGTACTGAAGTC -3′, RV 5′- GAGGAACGGTGACATGCTCAT -3′ Cyclin B2: FW 5′- CCGACGGTGTCCAGTGATTT -3′, RV 5′- TGTTGTTTTGGTGGGTTGAACT -3′ B-Myb: FW 5′- CCGGAGCAGAGGGATAGCA -3′, RV 5′- CAGTGCGGTTAGGGAAGTGG -3′ Ubiquitin: FW 5′- CACTTGGTCCTGCGCTTGA -3′, RV 5′- CAATTGGGAATGCAACAACTTTAT -3′. Purification of recombinant proteins GST-cyclin F and GST were expressed in Escherichia coli Rosetta (DE3) from the (pGEX) vectors using 0.2 mM of isopropyl-b- D -thiogalactoside for induction for 3 h at 37 °C. Harvested cells were lysed by sonication in 2 × PBS pH 7.4, 1% Triton X-100 and protease inhibitor tablets (Sigma). Following centrifugation at 20,000 g , the cleared lysates were incubated with glutathione–sepharose beads (GE Healthcare), washed with 50-column volumes of 2 × PBS pH 7.4, 1% Triton X-100 and eluted with 5-column volumes 50 mM Tris/HCl, pH 8.0 containing 10 mM reduced glutathione. The eluate was loaded onto a Sephacryl S-100 gel filtration column equilibrated with 2 × PBS. Fractions containing the pure protein were pooled and stored at 4 °C prior to use. In vitro transcription/translation of full-length human B-Myb FLAG-tagged human B-Myb was produced using the TnT Coupled reticulocyte Lysate Systems kit. We mixed 25 μl of Rabbit reticulocyte lysate, 2 μl of reaction buffer, 1 μl of T7 RNA polymerase, 1 μl of each amino-acid mixture minus leucine and amino-acid mixture minus methionine 1 mM, 2 μl RNase inhibitor 20 U μl −1 , 1 μg of FLAG-human B-Myb plasmid and addition of nuclease-free water to 50 μl. Samples were incubated at 30 °C for 90 min. GST-pull-down assay GST and GST-cyclin F were bound to 30 μl of glutathione beads at 4 °C for 1 h. The beads were centrifuged at 4,000 g for 1 min at 4 °C and washed with 1 ml 2 × PBS, pH 7.4, 1% Triton-X four times. The beads with GST-fusion proteins were resuspended in 490 μl of lysis buffer and 10 μl of in vitro translated FLAG-tagged human B-Myb during 2 h at 4 °C. Thereafter, the beads were again centrifuged at 4,000 g for 1 min at 4 °C and washed with 1 ml of lysis buffer four times. Subsequently, the proteins bound to the glutathione beads were eluted by boiling the samples at 94 °C for 5 min with 30 μl of 2 × Laemmli sample buffer. The mix was then briefly centrifuged and 25 μl of the supernatant were loaded on a 4–12% Tris-Bis NuPage gel. This was transferred to a nitrocellulose membrane. Immunoblotting was performed for cyclin F and GST. Ponceau S staining was employed to confirm equal protein loading in all samples. How to cite this article : Klein, D. K. et al . Cyclin F suppresses B-Myb activity to promote cell cycle checkpoint control. Nat. Commun. 6:5800 doi: 10.1038/ncomms6800 (2014).